Structural mechanisms of DIAP1 auto-inhibition and DIAP1-mediated inhibition of drICE The Drosophila inhibitor of apoptosis protein DIAP1 exists in an auto-inhibited conformation, unable to suppress the effector caspase drICE. Auto-inhibition is disabled by caspase-mediated cleavage of DIAP1 after Asp20. The cleaved DIAP1 binds to mature drICE, inhibits its protease activity, and, presumably, also targets drICE for ubiquitylation. DIAP1-mediated suppression of drICE is effectively antagonized by the pro-apoptotic proteins Reaper, Hid, and Grim (RHG). Despite rigorous effort, the molecular mechanisms behind these observations are enigmatic. Here we report a 2.4 Å crystal structure of uncleaved DIAP1–BIR1, which reveals how the amino-terminal sequences recognize a conserved surface groove in BIR1 to achieve auto-inhibition, and a 3.5 Å crystal structure of active drICE bound to cleaved DIAP1–BIR1, which provides a structural explanation to DIAP1-mediated inhibition of drICE. These structures and associated biochemical analyses, together with published reports, define the molecular determinants that govern the interplay among DIAP1, drICE and the RHG proteins. Caspases are the executioner of apoptosis in diverse organisms [1] . The initiator caspases are activated in response to upstream apoptotic signals and consequently activate the effector caspases, which inflict irreparable damage by cleaving a broad spectrum of cellular substrate proteins [2] , [3] . In mammals, the effector caspases-3 and -7 are activated by the initiator caspase-9. In Drosophila melanogaster , Dronc and drICE are the functional orthologs of caspase-9 and caspase-3, respectively. The activated caspases are subject to negative regulation by the inhibitor of apoptosis (IAP) proteins, exemplified by XIAP in mammals and DIAP1 in fruit flies [4] , [5] , [6] . IAPs suppress caspases either by direct inhibition of the protease activities [7] , [8] , [9] , [10] , or by ubiquitylation and presumably proteasome-mediated degradation [11] , [12] . Such negative regulation is countered by Smac/Diablo in mammals and RHG in fruit flies, which share a conserved tetrapeptide motif at their amino-termini [13] . This tetrapeptide binds a conserved surface groove on the BIR domains of IAPs and is known as the IAP-binding motif (IBM) [14] , [15] , [16] . Mutually exclusive binding to the BIR domains by IBMs present in either caspases or Smac/Diablo, and RHG is central for caspase regulation [5] , [13] . During homeostasis, the Dronc zymogen uses an internal peptide to recognize the conserved surface groove on the second BIR domain (BIR2) of DIAP1 (ref. 11 ). This interaction is required for the ubiquitylation of Dronc, mediated by the DIAP1–RING domain [11] , [12] . During apoptosis, the RHG proteins use their IBMs to bind the same surface groove [11] , hence releasing Dronc zymogen from DIAP1-mediated negative regulation. The freed Dronc zymogen is activated by the Dark apoptosome. In contrast to Dronc, the mechanism by which drICE is regulated by DIAP1, and RHG remains largely enigmatic, in part, owing to a complex network of interactions among these proteins. DIAP1 is both a substrate and a negative regulator of drICE. The full-length DIAP1 exists in an auto-inhibited conformation, exhibiting weak interactions with drICE and unable to inhibit the protease activity of drICE [17] , [18] . The mechanism of auto-inhibition was attributed to either intra-molecular interactions between the DIAP1 N-terminal sequences and the first BIR domain (BIR1) [17] or other yet-to-be-characterized interactions [18] . In either case, caspase-mediated cleavage of DIAP1 after Asp20 disables auto-inhibition, allowing DIAP1 to stably interact with and negatively regulate drICE [17] , [18] . The mechanism of drICE suppression was proposed to involve either direction inhibition of drICE protease activity by the cleaved DIAP1–BIR1 domain [17] or non-degradative polyubiquitylation of drICE by the RING domain [18] . Notably, polyubiquitylation of drICE was thought to ultimately result in the inhibition of drICE protease activity [18] . Further confounding the picture was the observation that cleavage of DIAP1 facilitated its degradation via the N-end rule pathway [19] . Regardless of how DIAP1 suppresses drICE, the RHG proteins antagonize DIAP1 function through direct interactions with its BIR1 and BIR2 domains [11] , [16] , [20] . In this study, we identify the molecular mechanisms for DIAP1 auto-inhibition and drICE inhibition by DIAP1–BIR1. Our studies serve as a framework for interpreting a body of published biological observations. Mechanism of auto-inhibition of the DIAP1–BIR1 domain We previously demonstrated that the DIAP1–BIR1 fragment 21–145, but not the uncleavable fragment 1–145 (D20A), potently inhibited the protease activity of drICE [17] . The N-terminal residue Met1 preceding Ala2 in DIAP1 is invariably removed during recombinant expression in Escherichia coli by bacterial methionine amino-peptidase, which is evolutionarily conserved across numerous organisms including fruit flies. The mutation A2M disabled auto-inhibition, allowing the resulting BIR1 fragment (1–145, D20A, A2M) to potently inhibit drICE [17] . These observations strongly suggest that the BIR1 domain of DIAP1 exists in an auto-inhibitory conformation, with its N-terminal amino acids, particularly Ala2, occupying a conserved groove on BIR1 (ref. 17 ). This intra-molecular interaction model is supported by gel filtration experiments, which rule out the possibility of inter-molecular interactions involving the N-terminal residues ( Supplementary Fig. S1a ). 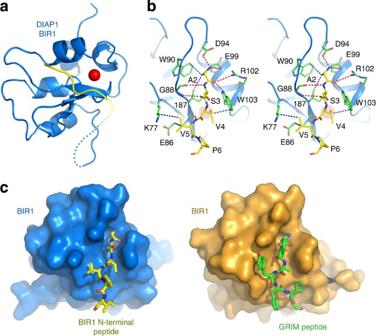Figure 1: Mechanism of auto-inhibition in the DIAP1–BIR1 domain. (a) Structure of the DIAP1–BIR1 domain in an auto-inhibited conformation. The N-terminal fragment is coloured yellow, and the zinc ion is represented by a red sphere. The disordered residues are indicated by a dotted line. (b) A stereo view of the specific interactions between the N-terminal amino acids and the conserved surface groove on the BIR1 domain. Hydrogen bonds and van der Waals contacts are represented by red and blue dashed lines, respectively. (c) Structural comparison of the auto-inhibited BIR1 (left panel) and the Grim–BIR1 complex (right panel, PDB accession code 1SEO17). Note the considerably more extensive interactions in the Grim–BIR1 interface. All structural images were generated using PyMol40. To conclusively corroborate this model, we crystallized the auto-inhibited DIAP1–BIR1 and determined its X-ray structure at 2.4 Å resolution ( Table 1 ; Fig. 1a ; Supplementary Fig. S1b ). Table 1 Statistics of data collection and refinement. Full size table Figure 1: Mechanism of auto-inhibition in the DIAP1–BIR1 domain. ( a ) Structure of the DIAP1–BIR1 domain in an auto-inhibited conformation. The N-terminal fragment is coloured yellow, and the zinc ion is represented by a red sphere. The disordered residues are indicated by a dotted line. ( b ) A stereo view of the specific interactions between the N-terminal amino acids and the conserved surface groove on the BIR1 domain. Hydrogen bonds and van der Waals contacts are represented by red and blue dashed lines, respectively. ( c ) Structural comparison of the auto-inhibited BIR1 (left panel) and the Grim–BIR1 complex (right panel, PDB accession code 1SEO [17] ). Note the considerably more extensive interactions in the Grim–BIR1 interface. All structural images were generated using PyMol [40] . Full size image As anticipated, the N-terminal sequence Ala2–Ser3–Val4–Val5 binds to the conserved surface groove ( Fig. 1a ). This interface comprises 7 hydrogen bonds (H-bonds) and a small number of van der Waals contacts, of which approximately half are mediated by the N-terminal residue Ala2 ( Fig. 1b ). The positively charged amino group of Ala2 donates two H-bonds to the negatively charged side chains of Asp94 and Glu99, whereas the carbonyl oxygen of Ala2 accepts two H-bonds from Arg102 and Trp103. The side chain of Ala2 is nestled in a hydrophobic pocket formed by Ile87, Trp90 and the aliphatic portion of Glu99 side chain. In addition, the main chain groups of Ser3 mediate two H-bonds to Gly88, and the amide nitrogen of Val5 hydrogen bonds to the carbonyl oxygen of Glu86. Val4 and Val5 also make some van der Waals contacts with surrounding amino acids. Together, these interactions allow the peptide-binding groove of BIR1 to be recognized by its own N-terminal sequences, amounting to auto-inhibition. This binding mode is reminiscent of the interactions between DIAP1–BIR1 and the RHG N-terminal peptides [17] ( Fig. 1c ; Supplementary Fig. S1c ). The key shared feature is the indispensable role of the N-terminal residue Ala. Another notable similarity is a pair of H-bonds mediated by the residue immediately following Ala, Ser3 in BIR1, Val3 in Reaper/Hid, and Ile3 in Grim. However, compared with the N-terminal peptide of DIAP1–BIR1, the N-terminal sequences of RHG have considerably more interactions with residues in the groove. In addition to 8 intermolecular H-bonds, the Grim peptide also makes extensive van der Waals contacts to hydrophobic residues in the BIR1 groove [17] ( Fig. 1c ; Supplementary Fig. S1c ). The buried surface area is approximately 833 Å 2 for the Grim–BIR1 interface and only 621 Å 2 for BIR1 auto-inhibition. Consistently, the isolated RHG peptides bind toDIAP1–BIR1 (residues 21–145) with dissociation constants of 0.12–0.76 μM [17] , whereas the free DIAP1 fragment 2–20 failed to form a stable complex with BIR1 (residues 21–145). Although the free DIAP1 fragment 2–20 does not stably interact with BIR1, the covalent linkage in the uncleaved DIAP1 greatly enhances the interactions by markedly increasing the local concentration of the N-terminal binding sequence towards the BIR1 domain. Cleavage of DIAP1 after Asp20, by drICE or other activated caspases, severs the covalent linkage, leading to dissociation of the N-terminal fragment 2–20 and loss of auto-inhibition. Characterization of drICE inhibition by BIR1 To elucidate the mechanism of drICE inhibition by DIAP1–BIR1, we attempted to crystallize a binary complex between BIR1 and the wild-type (WT), catalytically active drICE. Despite rigorous effort, we failed to generate any usable crystals. This problem might be due to flexible sequences in the surface of the BIR1–drICE complex that hinder crystal packing interactions. We sought to remedy this problem by biochemically identifying a minimalist BIR1–drICE complex. First, we examined the sequence requirement for drICE. The WT, mature drICE contains a large subunit (residues 29–232) and a small subunit (residues 233–339). The extended N-terminal fragment of drICE (29–83) is predicted to be highly hydrophilic. We attempted to shorten this sequence without affecting drICE protease activity. As previously reported [17] , the WT, mature drICE efficiently cleaved the substrate protein Dronc (C318A, F118E), and this activity was potently inhibited by DIAP1–BIR1 (residues 31–145) ( Fig. 2a ). Removal of residues 33–62 or 29–62 in drICE had no apparent impact on its protease activity; however, only drICE Δ33–62, but not Δ29–62, allowed efficient inhibition by BIR1 ( Fig. 2b , lanes 1–5). Similar conclusion was reached for drICE variants Δ33–77 and Δ29–77 ( Fig. 2b , lanes 6–9). We concluded that residues 33–77 are dispensable for the protease activity of drICE and the residues Ala29–Leu30–Gly31–Ser32 are indispensable for inhibition by DIAP1–BIR1. The latter conclusion confirms a previous report [21] . Notably, deletion of residues 33–82 or 29–82 in drICE negatively affected its protease activity ( Fig. 2b , lanes 10–13). Thus drICE Δ33–77 might represent an ideal construct for crystallization. 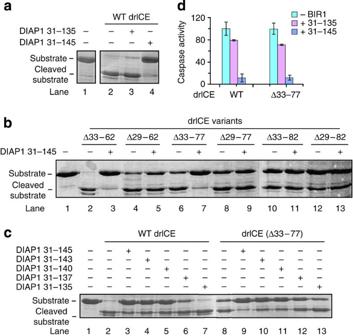Figure 2: Characterization of the BIR1–drICE interactions. (a) The WT, mature drICE is efficiently inhibited by DIAP1–BIR1 (residue 31–145), but not by BIR1 (residues 31–135) (lanes 1–4). Shown here in all three panels are representative SDS–PAGE gels stained by Coomassie blue. A catalytically inactive mutant of Dronc (C318A, F118E) was used as the substrate. (b) Identification of a minimalist drICE that retains the same protease activity and sensitivity to DIAP1–BIR1 as the WT drICE. Deletion of the amino acids 33–62 or 33–77 in drICE had no detectable effect on its protease activity or inhibition by DIAP1–BIR1 (lanes 1–3 and 6–7). Deletion of four additional residues 29–32 in drICE crippled its sensitivity to DIAP1–BIR1 (lanes 4–5 and 8–9), whereas removal of residues 78–82 compromised the protease activity (lanes 10–13). (c) Identification of a suitable DIAP1–BIR1 fragment for complex formation with drICE. Successive deletion of the C-terminal amino acids in DIAP1–BIR1 (residues 31–145) resulted in progressive loss of the ability to inhibit WT drICE (lanes 1–7) or the drICE variant Δ33–77 (lanes 8–13). (d) Comparison of WT drICE and the drICE variant used for crystallization (Δ33–77). The fluorogenic substrate Ac–DEVD–AMC was used as the substrate. Figure 2: Characterization of the BIR1–drICE interactions. ( a ) The WT, mature drICE is efficiently inhibited by DIAP1–BIR1 (residue 31–145), but not by BIR1 (residues 31–135) (lanes 1–4). Shown here in all three panels are representative SDS–PAGE gels stained by Coomassie blue. A catalytically inactive mutant of Dronc (C318A, F118E) was used as the substrate. ( b ) Identification of a minimalist drICE that retains the same protease activity and sensitivity to DIAP1–BIR1 as the WT drICE. Deletion of the amino acids 33–62 or 33–77 in drICE had no detectable effect on its protease activity or inhibition by DIAP1–BIR1 (lanes 1–3 and 6–7). Deletion of four additional residues 29–32 in drICE crippled its sensitivity to DIAP1–BIR1 (lanes 4–5 and 8–9), whereas removal of residues 78–82 compromised the protease activity (lanes 10–13). ( c ) Identification of a suitable DIAP1–BIR1 fragment for complex formation with drICE. Successive deletion of the C-terminal amino acids in DIAP1–BIR1 (residues 31–145) resulted in progressive loss of the ability to inhibit WT drICE (lanes 1–7) or the drICE variant Δ33–77 (lanes 8–13). ( d ) Comparison of WT drICE and the drICE variant used for crystallization (Δ33–77). The fluorogenic substrate Ac–DEVD–AMC was used as the substrate. Full size image Next, we examined the sequence requirement for DIAP1–BIR1. The BIR1 fragment 31–145, at a concentration of 5 μM, inhibited the protease activity of WT drICE by approximately 90 per cent ( Fig. 2c , lanes 1–3). BIR1 fragments with longer N-terminal extension exhibited a similar level of drICE inhibition. By contrast, deletion of amino acids from the carboxy-terminal end of BIR1 (residues 31–145) resulted in progressive loss of the ability to inhibit drICE. Notably, the BIR1 fragments 31–143 and 31–140, but not 31–137 or 31–135, potently inhibited the protease activity of drICE, suggesting direct involvement of residues 136–140 in binding to and/or inhibition of drICE ( Fig. 2c , lanes 4–7). Of all the BIR1 fragments tested, residues 31–145 appeared to most potently inhibit both WT and Δ33–77 drICE ( Fig. 2c ). Finally, the protease activities of WT and Δ33–77 drICE were nearly identical towards the fluorogenic substrate Ac–DEVD–AMC ( Fig. 2d ). The activities were inhibited to similar extents by the DIAP1–BIR1 fragment 31–145 but resisted inhibition by the fragment 31–135. Structure of a BIR1–drICE complex On the basis of biochemical characterization, we focused our crystallization effort on the minimalist complex between drICE Δ33–77 and DIAP1–BIR1 31–145. We generated crystals in the space group I2 1 2 1 2 1 . These crystals diffracted X-rays to a resolution limit of 10 Å. Dehydration and repeated annealing of the crystals markedly improved the X-ray diffraction limit. Eventually, we solved the structure at 3.5 Å resolution by molecular replacement ( Table 1 ; Fig. 3a ). In each asymmetric unit, two molecules of BIR1 bind a homo-dimer of drICE, forming a roughly symmetric hetero-tetramer ( Fig. 3a ). To facilitate structural interpretation, we also crystallized free drICE and solved its structure at 2.7 Å resolution ( Table 1 ; Fig. 3b ). 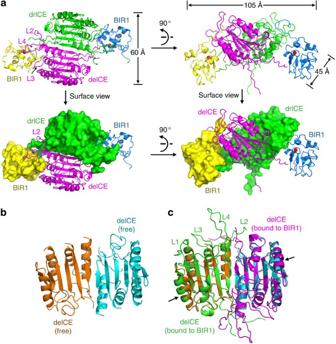Figure 3: Crystal structures of drICE in isolation and in complex with DIAP1–BIR1. (a) Overall structure of the catalytically active drICE variant (Δ33–77) bound to the BIR1 domain (residues 31–145) of DIAP1. A drICE homo-dimer, with two protomers coloured green and magenta, is recognized by two molecules of DIAP1–BIR1 (shown in yellow and blue). Two perpendicular views, along with their surface representation, are shown to highlight the overall features of the hetero-tetrameric complex. Each BIR1 molecule interacts with both protomers of drICE. This colouring scheme is preserved in panelcandFigure 4. (b) Overall structure of a free, catalytically active drICE. The two protomers are coloured cyan and orange. The four active site loops, L1 through L4, are largely disordered in the crystals and not shown here. (c) Structural overlay of free drICE with BIR1-bound drICE. The active site loops have well-defined conformation only in the BIR1-bound drICE. Figure 3: Crystal structures of drICE in isolation and in complex with DIAP1–BIR1. ( a ) Overall structure of the catalytically active drICE variant (Δ33–77) bound to the BIR1 domain (residues 31–145) of DIAP1. A drICE homo-dimer, with two protomers coloured green and magenta, is recognized by two molecules of DIAP1–BIR1 (shown in yellow and blue). Two perpendicular views, along with their surface representation, are shown to highlight the overall features of the hetero-tetrameric complex. Each BIR1 molecule interacts with both protomers of drICE. 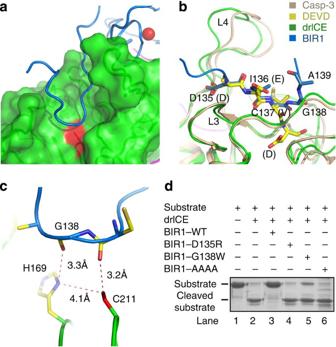Figure 4: Mechanism of drICE inhibition by the DIAP1–BIR1 domain. (a) A close-up view of the substrate-binding groove of drICE occupied by a C-terminal fragment of DIAP–BIR1 (residues 135–141). drICE is shown in surface representation (green) and BIR1 is coloured blue. (b) The DIAP1 residues 135–141 spatially overlap with the binding site for caspase substrate/inhibitor. The main chain atoms of Asp135–Ile136–Cys137 nearly coincide with those of the first three amino acids Asp–Glu–Val of the inhibitor DEVD–CHO. (c) The DIAP1 fragment 135–141 is not a substrate of drICE. The catalytic residue of drICE, Cys211, donates a H-bond to the carbonyl oxygen atom of Cys137 in the DIAP1 fragment. This interaction, together with a second H-bond between His169 and the carbonyl oxygen atom of Gly138 in DIAP1, prevents activation of the catalytic residue Cys211 and keeps it away from the nearest peptide bond between Cys137 and Gly138 in the DIAP1 fragment. (d) Mutation of Asp135–Ile136–Cys137–Gly138 in DIAP1–BIR1 led to loss of its ability to inhibit the protease activity of drICE. Whereas the presence of 10 μM WT DIAP1–BIR1 led to complete inhibition of drICE activity (lane 3), similar amounts of BIR1–D135R, G138W, or AICG-to-AAAA, failed to inhibit drICE activity (lanes 4–6). This colouring scheme is preserved in panel c and Figure 4 . ( b ) Overall structure of a free, catalytically active drICE. The two protomers are coloured cyan and orange. The four active site loops, L1 through L4, are largely disordered in the crystals and not shown here. ( c ) Structural overlay of free drICE with BIR1-bound drICE. The active site loops have well-defined conformation only in the BIR1-bound drICE. Full size image Structure of the BIR1–drICE hetero-tetramer measures ∼ 105 Å in length, 60 Å in width, and 45 Å in thickness ( Fig. 3a ). Most notably, each BIR1 domain interacts with both protomers of the drICE homo-dimer. Each BIR1 domain sits above the active site of a drICE protomer, with its C-terminal fragment (residues 130–145) occupying the substrate-binding groove of the same drICE protomer. The conserved peptide-binding groove of this BIR1 domain receives the N-terminal sequences Ala29–Leu30–Gly31–Ser32 from the adjacent drICE protomer ( Fig. 3a ). This structural observation provides an immediate clue to two questions: how drICE is inhibited by DIAP1–BIR1 and why the N-terminal sequences of drICE are required for binding to DIAP1–BIR1. The observed binding mode also provides a preliminary explanation to the puzzle of why deletion of residues 136–145 in the BIR1 domain abrogated its ability to inhibit drICE. The interaction between the C-terminal fragment of BIR1 and the active-site groove of drICE is buttressed by another interface between the backside of the L4 loop and BIR1. Together, these interactions involve a buried surface area of ∼ 2,208 Å 2 . In the BIR1–drICE structure, all four active-site loops L1–L4 adopt well-defined conformations ( Fig. 3a ). These loops are directly involved in interactions with BIR1. By contrast, these loops exhibited no apparent electron density in the structure of free drICE ( Fig. 3b,c ). Presumably, these loops are flexible in free drICE and become ordered upon binding to BIR1. The conformational differences between free and BIR1-bound drICE is reminiscent of those between free and inhibitor-bound caspase-7 (refs 22 , 23 ). Mechanism of drICE inhibition by BIR1 DIAP1 employs a short peptide fragment (residues 135–141) to recognize the active site of drICE ( Fig. 4a ). In the BIR1–drICE complex, DIAP1 residues 135–141 spatially overlap with the binding site for caspase substrate. Strikingly, the main chain atoms of DIAP1 Asp135–Ile136–Cys137 almost exactly coincide with those of the first three amino acids Asp–Glu–Val of the inhibitor DEVD–CHO ( Fig. 4b ; Supplementary Fig. S2a ). Thus DIAP1 inhibits drICE by blocking substrate entry. Why does drICE not cleave the DIAP1 fragment 135–141? The answer lies in the specific conformation of the DIAP1 fragment and its interactions with surrounding amino acids in drICE ( Fig. 4c ; Supplementary Fig. S2b ). The catalytic residue of drICE, Cys211, donates a H-bond to the carbonyl oxygen atom of Cys137 in the DIAP1 fragment. This interaction, together with a second H-bond between His169 and carbonyl oxygen of Gly138 in DIAP1, appears to block activation of the catalytic residue Cys211 and keeps it away from the nearest peptide bond between Cys137 and Gly138 in the DIAP1 fragment. Figure 4: Mechanism of drICE inhibition by the DIAP1–BIR1 domain. ( a ) A close-up view of the substrate-binding groove of drICE occupied by a C-terminal fragment of DIAP–BIR1 (residues 135–141). drICE is shown in surface representation (green) and BIR1 is coloured blue. ( b ) The DIAP1 residues 135–141 spatially overlap with the binding site for caspase substrate/inhibitor. The main chain atoms of Asp135–Ile136–Cys137 nearly coincide with those of the first three amino acids Asp–Glu–Val of the inhibitor DEVD–CHO. ( c ) The DIAP1 fragment 135–141 is not a substrate of drICE. The catalytic residue of drICE, Cys211, donates a H-bond to the carbonyl oxygen atom of Cys137 in the DIAP1 fragment. This interaction, together with a second H-bond between His169 and the carbonyl oxygen atom of Gly138 in DIAP1, prevents activation of the catalytic residue Cys211 and keeps it away from the nearest peptide bond between Cys137 and Gly138 in the DIAP1 fragment. ( d ) Mutation of Asp135–Ile136–Cys137–Gly138 in DIAP1–BIR1 led to loss of its ability to inhibit the protease activity of drICE. Whereas the presence of 10 μM WT DIAP1–BIR1 led to complete inhibition of drICE activity (lane 3), similar amounts of BIR1–D135R, G138W, or AICG-to-AAAA, failed to inhibit drICE activity (lanes 4–6). Full size image To examine the sequence requirement for the inhibition of drICE, we generated three BIR1 variants targeting the sequence Asp135–Ile136–Cys137–Gly138. The missense mutation D135R and the quadruple mutation AICG-to-AAAA both led to complete abrogation of BIR1-mediated inhibition of drICE ( Fig. 4d ). The mutation G138W also severely compromised drICE inhibition ( Fig. 4d ). Interactions between BIR1 and drICE There are three discrete interfaces between BIR1 and drICE ( Fig. 5a ). The active site of drICE contains 6 intermolecular H-bonds and a number of van der Waals contacts ( Fig. 5b ; Supplementary Fig. S3a ). Notably, 3 of the 6 H-bonds only involve main chain atoms, between BIR1–Tyr134/Ile136 and drICE–Thr261/Arg259. The carboxylate side chain of BIR1–Asp141 accepts a H-bond from the ɛ-amine group of drICE–Lys110. These H-bonds are reinforced by van der Waals interactions between BIR1 Ile136–Cys137–Gly138–Ala139 and the surrounding drICE residues His169, Cys 211, Tyr256, Trp258 and Arg259. The conformation of BIR1 135–141 is further stabilized by three intra-molecular H-bonds between Asp135 and Arg111. 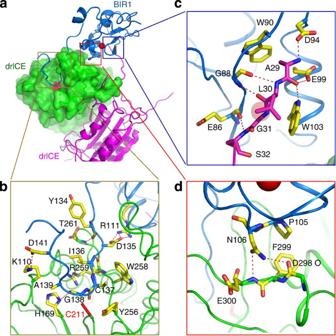Figure 5: Interactions between DIAP1–BIR1 and drICE. (a) The interactions between drICE and BIR1 constitute three distinct interfaces, of which two involve peptide–protein interactions and only one involves protein–protein interface. (b) A close-up view of the interface between the C-terminal sequences of the BIR1 domain and the active site of drICE. A number of BIR1 residues are positioned in close proximity to the catalytic residue Cys211 of drICE, blocking substrate access. (c) A close-up view of the interface between the N-terminal sequences ALGS of drICE and the BIR1 domain. Hydrogen bonds are represented by red dashed lines. The interactions closely resemble those in the auto-inhibited BIR1 domain, with the N-terminal Ala residue playing a dominant role at this interface. (d) A close-up view of the protein–protein interface between BIR1 and drICE. This interface is mediated by Pro105 and Asn106 of DIAP1. Figure 5: Interactions between DIAP1–BIR1 and drICE. ( a ) The interactions between drICE and BIR1 constitute three distinct interfaces, of which two involve peptide–protein interactions and only one involves protein–protein interface. ( b ) A close-up view of the interface between the C-terminal sequences of the BIR1 domain and the active site of drICE. A number of BIR1 residues are positioned in close proximity to the catalytic residue Cys211 of drICE, blocking substrate access. ( c ) A close-up view of the interface between the N-terminal sequences ALGS of drICE and the BIR1 domain. Hydrogen bonds are represented by red dashed lines. The interactions closely resemble those in the auto-inhibited BIR1 domain, with the N-terminal Ala residue playing a dominant role at this interface. ( d ) A close-up view of the protein–protein interface between BIR1 and drICE. This interface is mediated by Pro105 and Asn106 of DIAP1. Full size image The peptide-binding groove of BIR1 is recognized by the N-terminal tetrapeptide Ala29–Leu30–Gly31–Ser32 of the adjacent drICE protomer ( Fig. 5c ; Supplementary Fig. S3b ). At this interface, Ala29 has a pivotal role by making three H-bonds and a number of van der Waals contacts. These interactions closely resemble those observed in the structure of auto-inhibited BIR1 domain ( Fig. 1 ). Together, these observations provide a satisfactory explanation to the questions of why auto-inhibited BIR1 exhibits no inhibition of drICE and why deletion of the tetrapeptide Ala29–Leu30–Gly31–Ser32 in drICE no longer allows BIR1-mediated inhibition. Formation of the BIR1–drICE complex is further augmented by a protein–protein interface, involving BIR1 residues Pro105 and Asn106, which interact with the L4 loop of drICE ( Fig. 5d ; Supplementary Fig. S3c ). A weak DIAP1 gain-of-function mutation, P105S (ref. 24 ), maps to this interface. Although the consequence of this mutation is not severe enough to abolish the interaction between drICE and DIAP1 (ref. 17 ), it likely weakens the association. Biological implication Our structural observations provide a framework for understanding a body of developmental observations. A number of DIAP1 gain-of-function mutations were mapped to the BIR1 domain, which could suppress RHG-induced apoptosis [24] , [25] . Two of these mutations, G88S and G88D (ref. 24 ), affect the same amino acid in the peptide-binding groove of DIAP1–BIR1. Among the three interfaces between BIR1 and drICE, only one (involving the peptide-binding groove) is affected by these mutations ( Fig. 5c ). Thus the mutant DIAP1 proteins might still remain associated with drICE, which was biochemically verified [17] . By contrast, because BIR1 binding by RHG relies primarily on the integrity of the peptide-binding groove, these mutations may have a deleterious consequence, evicting the P4 residue from RHG and disallowing stable interactions between BIR1 and RHG [17] . N117K is a loss-of-function mutation that enhanced RHG-induced cell death [24] . In the crystal structure, Asn117 accepts a H-bond from Arg47, which nucleates four H-bonds to stabilize the overall conformation ( Supplementary Fig. 4a ). Mutation of Asn117 to Lys is predicted to disrupt the interaction with Arg47 and negatively affect the conformation of BIR1, particularly the C-terminal fragment. These changes, in turn, likely weaken the association between DIAP1 and drICE [20] . In the structure of drICE, Asn116 has a structural role by mediating a network of H-bonds with Glu102 of the L1 loop and Lys137 ( Supplementary Fig. 4b ). Mutation of Asn116 to Tyr is predicted to disrupt these interactions, compromising the stability of drICE and perhaps altering the conformation of the active site. This structural analysis provides a plausible explanation to the observation that the mutation N116Y resulted in accelerated degradation and loss-of-function for drICE [26] . DIAP1-mediated ubiquitylation of drICE was recently found to result in inhibition of its protease activity, but not proteasomal degradation [18] . The mechanism was attributed to steric hindrance with substrate entry. Examination of the drICE structure reveals that the only Lys residue that may pose steric hindrance to substrate entry is Lys110 ( Supplementary Fig. 5 ). However, the variant drICE–K110R appeared to be susceptible to DIAP1 suppression [18] . Strikingly, all 9 Lys residues in drICE had to be replaced by Arg for drICE to be resistant to DIAP1 suppression [18] . Structural analysis failed to identify an obvious basis for this finding. Detailed biochemical characterization may be needed to further evaluate the mechanism by which ubiquitylation regulates drICE activity. The structural and biochemical information presented in this study, together with findings reported elsewhere [11] , [12] , [17] , [18] , gives rise to a model on the interplay of Dronc, drICE, DIAP1, and the RHG proteins ( Fig. 6 ). During homeostasis, DIAP1 targets the Dronc zymogen for ubiquitylation and presumably proteasome-mediated degradation. This regulation depends on the interaction between a peptide fragment of Dronc and the conserved groove on DIAP1–BIR2 (ref. 11 ). DIAP1 exists in an auto-inhibited conformation. Caspase-mediated cleavage of DIAP1 after Asp20 disables auto-inhibition, allowing the resulting DIAP1 fragment to bind to and inhibit active drICE. During apoptosis, the RHG proteins use their N-terminal peptides to compete with drICE and Dronc for binding to the conserved peptide-binding grooves on the BIR1 and BIR2 domains, respectively. Such competition results in the release of drICE and Dronc from DIAP1. The freed Dronc zymogen is activated by the Dark apoptosome and the mature Dronc cleaves and activates drICE. In this regard, drICE, DIAP1 and the RHG proteins together provide a fail-safe mechanism to ensure appropriate drICE activation only under bona fide apoptotic conditions. 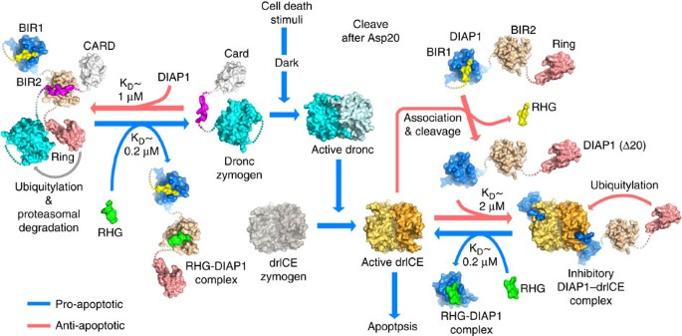Figure 6: A mechanistic model on the interplay of apoptotic caspases and their regulators inDrosophila. In non-apoptotic cells, DIAP1 interacts with Dronc and keeps its level low through ubiquitylation. drICE exists in an auto-inhibited conformation. In apoptotic cells, the RHG proteins compete with Dronc for binding to the same surface groove on the BIR2 domain of DIAP1, hence disabling DIAP1-mediated ubiquitylation of Dronc. The mature Dronc no longer interacts with and hence is no longer regulated by DIAP1. Dronc activates effector caspases such as drICE, which cleaves DIAP1 after Asp20. This cleavage disables the auto-inhibition of DIAP1, allowing the BIR1 domain to inhibit the protease activity of drICE. The negative regulation of drICE by the cleaved DIAP1 may represent a fail-safe mechanism for cells to guard against unwanted cell death. The cleaved DIAP1 may also ubiquitylate drICE, which also led to its inhibition. Under the unmistaken conditions of cell death, the RHG proteins relieve drICE inhibition by competing with drICE for binding to DIAP1–BIR1, thus allowing the freed drICE to cleave a broader spectrum of substrate proteins, inducing cell death. Figure 6: A mechanistic model on the interplay of apoptotic caspases and their regulators in Drosophila . In non-apoptotic cells, DIAP1 interacts with Dronc and keeps its level low through ubiquitylation. drICE exists in an auto-inhibited conformation. In apoptotic cells, the RHG proteins compete with Dronc for binding to the same surface groove on the BIR2 domain of DIAP1, hence disabling DIAP1-mediated ubiquitylation of Dronc. The mature Dronc no longer interacts with and hence is no longer regulated by DIAP1. Dronc activates effector caspases such as drICE, which cleaves DIAP1 after Asp20. This cleavage disables the auto-inhibition of DIAP1, allowing the BIR1 domain to inhibit the protease activity of drICE. The negative regulation of drICE by the cleaved DIAP1 may represent a fail-safe mechanism for cells to guard against unwanted cell death. The cleaved DIAP1 may also ubiquitylate drICE, which also led to its inhibition. Under the unmistaken conditions of cell death, the RHG proteins relieve drICE inhibition by competing with drICE for binding to DIAP1–BIR1, thus allowing the freed drICE to cleave a broader spectrum of substrate proteins, inducing cell death. Full size image The underpinning of this regulatory network is competition among multiple protein–protein interactions mediated by the conserved grooves of the BIR1 and BIR2 domains of DIAP1. Auto-inhibition of DIAP1–BIR1 is achieved by occupation of this groove by its own N-terminal sequence ASVV. The free peptide ASVV does not stably associate with BIR1; the covalent linkage facilitates the binding by increasing the local concentration of ASVV. This binding arrangement allows disabling of auto-inhibition upon cleavage of DIAP1 after Asp20. Inhibition of drICE by BIR1 requires occupation of this groove by the N-terminal sequences ALGS of drICE. Similar to ASVV, the free ALGS peptide exhibited no detectable binding to the BIR1 fragment 21–145. Three weak interfaces between BIR1 and drICE cooperate to yield a stable hetero-tetramer with a K D of approximately 1–2 μM. Removal of drICE inhibition by BIR1 depends on the interactions between RHG and the peptide-binding groove, with K D values of 0.12–0.76 μM (ref. 17 ). Endowing RHG with the strongest interactions ensures an apoptotic phenotype once the RHG proteins are activated in cells. We acknowledge that the proposed model may be simplistic, as the network of protein–protein interactions and regulation is likely to be more complex in vivo . Nevertheless, the biophysical underpinnings described in this model are likely to have a role in various stages of apoptosis regulation. An IAP-binding motif, though not ostensibly abbreviated as IBM, was originally defined to contain four contiguous amino acids that resemble the Smac tetrapeptide AVPI [14] , [15] , [16] . This structurally defined motif, with binding affinities of 0.1–1 μM, has stringent requirement for the first (P1), third (P3) and fourth (P4) amino acids [13] . The P1 residue must be Ala, which binds to a small hydrophobic pocket on one end of the conserved groove on BIR domain. The P4 residue must be hydrophobic, preferably bulky, to occupy a greasy pocket on the other end of the groove. Deletion of P1 or P4 in a tetrapeptide results in abrogation of stable interaction with the BIR domain. The P3 residue is either Pro or Ala. Pro as P3, with its unique backbone configuration, optimizes simultaneous binding by both P1 and P4 residues for DIAP1–BIR2 or XIAP–BIR3. Ala as P3 can be better accommodated by DIAP1–BIR1 and XIAP–BIR2. In recent studies [18] , [21] , IBM was redefined to contain three contiguous amino acids, with P3 no longer restricted to Pro or Ala. Such tripeptides, ALG/AKG for drICE/Dcp1, or their longer variants, ALGS/AKGC for drICE/Dcp1, do not meet the structural criteria for IBM. Importantly, these peptides in isolation do not form a stable complex with any BIR domain. The definition of such motifs as IBMs insinuates the incorrect assumption that such free peptide motifs may stably interact with the BIR domain. This assumption, in turn, has engendered ample confusion in data interpretation in recent years. An IBM at the N-terminus of the caspase-9 small subunit recognizes a conserved surface groove on XIAP–BIR3 (ref. 7 ); this interaction locks caspase-9 in the inhibited state. During apoptosis, Smac/Diablo uses a similar tetrapeptide motif to occupy the BIR3 groove, hence releasing caspase-9 and relieving XIAP-mediated inhibition [14] , [15] , [27] . Caspase-3 or -7 is inhibited by an 18-residue peptide segment preceding the BIR2 domain of XIAP [8] , [9] , [10] , [28] . Because both caspase-3 and drICE are inhibited directly at the active sites by XIAP and DIAP1, respectively, the overall appearance of the two BIR-caspase complexes is similar ( Supplementary Fig. S6a ). It should be noted, however, that the essential interactions and key features are quite different. For example, caspase-3 or -7 can be inhibited by an isolated 18-residue peptide fused to GST; but the intact BIR1 domain of DIAP1 is absolutely required for drICE inhibition. The orientation of the BIR domain relative to the caspase is different by approximately 90 degrees between caspase-3/BIR2 and drICE/BIR1 ( Supplementary Fig. S6b ). Importantly, the peptide-binding groove of XIAP–BIR2 does not have an apparent role in the inhibition of caspase-3 and -7. Using purified, recombinant proteins, we showed that the BIR1 domain of DIAP1 only forms a stable complex with active drICE following caspase-mediated cleavage of DIAP1 after Asp20 (ref. 17 ). The uncleaved DIAP1–BIR1 exhibited very weak binding to drICE. These observations contrast the report that both uncleaved and cleaved DIAP1–BIR1 bound to drICE similarly using coimmunoprecipitation [21] . The cleaved DIAP1, but not the uncleaved DIAP1, potently inhibits the proteolytic activity of drICE towards both peptide and protein substrates [17] . These observations unambiguously demonstrate that drICE sequestered by cleaved DIAP1 remains catalytically inactive. In fact, the conclusion that DIAP1-sequestered drICE was catalytically active, as reported by Tenev et al . contradicted their own biochemical observation that no protease activity was detectable towards peptide or protein substrate [21] . It is not uncommon for a substrate to be converted into a protease inhibitor upon cleavage, as exemplified by the pan-caspase inhibitor p35 (refs 29 , 30 ). The key question is not whether BIR1 inhibits drICE, but why BIR1-sequestered drICE continues to exhibit proteolytic activity towards the uncleaved DIAP1(refs 17 , 21 ). A time course analysis of DIAP1 cleavage shows that the protease activity of drICE was slowed down considerably over time, as the concentration of inhibitor—cleaved DIAP1—increased [17] . The level of drICE activity at the 15-minute time point was at least 6-fold higher than that at 90-minute point [17] . This observation again illustrates that the cleaved DIAP1 is a bona fide inhibitor of drICE. Some of the contrasting claims about the regulation of drICE by DIAP1 might be attributable to the limitations of the investigative methods. Biochemical and biophysical investigations, employing homogeneous, recombinant proteins, usually provide mechanistic answers to questions that pertain to protein–protein interactions and enzyme activities. The caveat, however, is whether such observations are biologically relevant, and if yes, to what extent these findings are important. By contrast, investigation by cellular biochemistry, exemplified by coimmunoprecipitation, provides important clues to molecular mechanisms. For both approaches, caution must be exercised for the interpretation of results. Notably, in some cases, the contrasting claims can be reconciled by a complex system. For example, despite our structural data demonstrating that the auto-inhibition of DIAP1 involves the binding of its N-terminal sequences to the BIR1 domain, it remains theoretically possible that additional interactions between the N- and C-terminal domains of DIAP1 may contribute to its auto-inhibition [18] . The best example is Apaf-1, whose auto-inhibition entails two elements: one by the C-terminal WD40 repeats and the other within the N-terminal half. Binding to cytochrome c relieves the auto-inhibition by the WD40 repeats [31] , and exchange of ADP for ATP defeats the auto-inhibition imposed by intra-domain interactions within the N-terminal-half [32] , [33] . Protein preparation To understand the auto-inhibition of DIAP1, we ligated the DIAP1 fragment 1–135 into the NdeI and XhoI sites of pET21b (Novagen). To improve the chance of crystallization, we deleted the flexible residues 6–12 and mutated a surface-exposed Cys residue, Cys89, to Ser in the DIAP1 fragment. For BIR1–drICE complex crystallization, a BIR1 construct containing residues 31–145 with C89S mutation was cloned into pET-15b (Novagen). The drICE variant Δ33–77 was cloned into pBB75. To obtain a stoichiometric complex between BIR1 and drICE, they were co-expressed in the bacterial strain BL21 (DE3). Expression of auto-inhibited BIR1 and BIR1–drICE complex was induced in LB medium with 0.2 mM isopropyl-β- D -thiogalactopyranoside at OD600 of 1.2 at 22 °C for 12 hours. Cells were resuspended in a buffer containing 25 mM Tris (pH 8.0) and 150 mM NaCl, and lysed using sonication. Following another centrifugation step, the supernatant was loaded to Ni 2+ +-NTA resin (Qiagen). The auto-inhibited BIR1 protein was eluted in a buffer containing 25 mM Tris, pH 8.0, 250 mM imidazole. The eluted protein was applied to Source-15Q (GE Healthcare) and the peak fraction was collected for crystallization. The complex protein was released from the column by thrombin cleavage for 4 hours at room temperature in a buffer containing 25 mM Tris (pH 8.0) and 150 mM NaCl. The protein was applied to Source-15Q (GE Healthcare) and the peak fraction was collected for cleavage by the wild-type Dronc protease at 18 °C overnight. After cleavage, the protein was concentrated to ∼ 25 mg ml −1 and applied to Superdex-200 (GE Healthcare) in a buffer containing 10 mM HEPES, pH 7.5, 100 mM NaCl, and 2 mM DTT. The peak fraction was collected for crystallization. WT drICE and Dronc were cloned into pBB75 with a C-terminal 6-Histidine-tag. The expression and purification of WT drICE and Dronc were the same as for DIAP1–BIR1. All point mutations were generated using a standard PCR-based cloning strategy. The expression and purification of WT drICE, Dronc, and all mutant proteins were the same as for DIAP1–BIR1. In vitro drICE assay In assays throughout this study, all recombinant proteins were purified to greater than 98% homogeneity. To ensure a uniform standard, all SDS–PAGE gels shown in this study were visualized by Coomassie blue staining. Reactions were carried out at 37 °C in an assay buffer containing 25 mM HEPES, pH7.5, 150 mM NaCl, and 2 mM DTT, for 60 min. Approximately 20 μg substrate (Dronc-C318A F118E) and 100 ng active drICE were used for each reaction. Fluorogenic assay for drICE The fluorogenic peptide Ac–DEVD–AMC was used as the substrate to measure the caspase activity of drICE variants. 50 μM substrate was used for each assay in the buffer containing 25 mM HEPE, pH 7.5, and 150 mM NaCl. Crystallization All of the crystals were grown at 18 °C by the hanging-drop vapour-diffusion method. Well buffer of auto-inhibited BIR1 contained 100 mM Bis-Tris, pH 5.4, 0.2 M (NH 4 ) 2 SO 4 , 3% (v/v) CH 3 OH, and 22% (wt/v) Polyethylene Glycol 3350 (Fluka). Well buffer of drICE contained 0.1M acetate, pH4.4, and 1.0 M (NH 4 ) 2 SO 4 . Well buffer of the BIR1-drICE complex contained 0.1 M Hepes, pH7.0, 0.3 M (NH 4 ) 2 SO 4 and 20% (w/v) Polyethylene Glycol 3350 (Fluka). All crystals grew to full sizes in about 2–7 days. But the BIR1–drICE crystals showed almost no diffraction. To optimize the crystals, we transferred the crystals to 4 °C cold room for 1 day, which improved the diffraction limit to about 7 A. Dehydration was used for optimization, and the final dehydration buffer contained 0.1 M Hepes, pH7.0, 0.3 M (NH 4 ) 2 SO 4 , 20% (w/v) Polyethylene Glycol 3350 (Fluka), and 20% (v/v) Polyethylene Glycol 400 (Fluka). Data collection and structural determination The diffraction images of free drICE, auto-inhibited BIR1, and the BIR1–drICE complex crystals were collected at the beamlines BL38B1 (SPring-8), BL41XU (SPring-8), and BL17U (SSRF), respectively. All data were integrated and scaled using the HKL2000 package [34] . Further processing was carried out using programs from the CCP4 suite [35] . Data collection statistics are summarized in Table 1 . The structure of free drICE was determined by molecular replacement method with the procaspase-7 (PDB accession code 1K88 (ref. 23 )) as the search model using PHASER [36] . The auto-inhibited BIR1 structure was solved with the DIAP1–BIR1 (PDB accession code 1SDZ (ref. 17 )). Structure of the BIR1–drICE complex was solved with the above drICE and BIR1 structures. The twinned structures of free drICE and auto-inhibited BIR1 were refined with REFMAC5 (ref. 37 ). In particular, the free drICE crystals displayed merohedral twinning. There are four macroscopic drICE molecules in the crystal, which are related by (H, K, L)/(−H, H+K, −L)/(−H, −K, L)/(K, H, −L) with the twinning fractions of 0.317, 0.181, 0.305, 0.196, respectively. The BIR1–drICE complex structure was refined using the program PHENIX [38] . The manual model modification was performed in COOT [39] . Accession codes: The atomic coordinates of the auto-inhibited BIR1, the BIR1-drICE complex, and the free drICE have been deposited in the Protein Data Bank with the accession codes 3SIQ , 3SIP , and 3SIR , respectively. How to cite this article: Li, X. et al . Structural mechanisms of DIAP1 auto-inhibition and DIAP1-mediated inhibition of drICE. Nat. Commun. 2:408 doi: 10.1038/ncomms1418 (2011).